iPSC-derived neural precursors exert a neuroprotective role in immune-mediated demyelination via the secretion of LIF The possibility of generating neural stem/precursor cells (NPCs) from induced pluripotent stem cells (iPSCs) has opened a new avenue of research that might nurture bench-to-bedside translation of cell transplantation protocols in central nervous system myelin disorders. Here we show that mouse iPSC-derived NPCs (miPSC-NPCs)—when intrathecally transplanted after disease onset—ameliorate clinical and pathological features of experimental autoimmune encephalomyelitis, an animal model of multiple sclerosis. Transplanted miPSC-NPCs exert the neuroprotective effect not through cell replacement, but through the secretion of leukaemia inhibitory factor that promotes survival, differentiation and the remyelination capacity of both endogenous oligodendrocyte precursors and mature oligodendrocytes. The early preservation of tissue integrity limits blood–brain barrier damage and central nervous system infiltration of blood-borne encephalitogenic leukocytes, ultimately responsible for demyelination and axonal damage. While proposing a novel mechanism of action, our results further expand the therapeutic potential of NPCs derived from iPSCs in myelin disorders. The development of cell-based therapies aimed at promoting remyelination in patients suffering from myelin disorders has been pursued in the last 30 years [1] , [2] . Although successful in supporting site-specific repair in focal myelin disease [3] , most of these cell-based therapeutic approaches have been mostly unsuccessful in multifocal inflammatory demyelinating diseases of the central nervous system (CNS), such as multiple sclerosis (MS). The recent demonstration that neural stem/precursor cell (NPCs)-based therapies can promote neuroprotection in experimental models of MS not only via cell replacement but also by secreting neuroprotective molecules—the so called bystander effect [4] , [5] , [6] , [7] — has suggested that such cells might represent in the near future a plausible alternative cell source for cell-based therapeutic strategy in MS. However, bench-to-bedside translation of NPC-based therapies in MS is still hampered by the allogenic nature of the so far only available source of NPCs for human trials. Indeed, although capable of promoting neuroprotection in a non-human primate model of MS [8] , fetal-derived NPCs do require concomitant immunosuppression when transplanted in humans. Induced pluripotent stem cells (iPSCs)—a new source of pluripotent stem cells obtained by genetic reprogramming of somatic cells [9] , [10] , [11] — might represent the ideal autologous source of NPCs for transplantation and translational purposes in MS. However, although the ability of iPSC-derived myelin-forming cells (for example, OPCs) to remyelinate congenitally demyelinated mice has been recently shown [3] , nothing is known about the capacity of these cells to protect neural tissue once transplanted in an hostile inflammatory demyelinated environment such as that characterizing MS. Here we show that mouse iPSC-derived NPCs (thereafter referred as miPSC-NPCs)—when intrathecally transplanted after disease onset in mice with experimental autoimmune encephalomyelitis (EAE), an animal model of MS—ameliorate clinical and pathological features of the disease. Transplanted miPSC-NPCs exert a neuroprotective effect in EAE not by differentiating into myelin producing cells but via the secretion of a specific neurotrophin, that is, leukaemia inhibitory factor (LIF), able to support the in vivo survival and differentiation of resident oligodendrocytes. This neuroprotective effect is, in turn, sufficient to limit the CNS-confined inflammatory process and the extent of the tissue damage. Generation of miPSCs from Sox2βGeo mouse fibroblasts Mouse embryonic fibroblasts (MEFs) were isolated from E14.5 Sox2βGeo knock-in E14.5 C57Bl/6 Sox2 βgeo/βgeo knock-in mouse embryos [12] and transduced with a lentiviral vector encoding for the Oct4, Sox2 and Klf4 transcription factors. miPSCs derived from the reprogramming of Sox2βGeo MEFs ( Fig. 1a ) express a βgeo cassette under the control of Sox2 promoter that gives cell resistance to neomycin and the ability to be recognized by X-gal staining ( Fig. 1b ). Five days after transduction, cells were harvested and plated onto Mitomycin C-treated MEF feeder cells. Thirty days later, some flat and round colonies were observed ( Fig. 1a ). miPSC colonies were picked based on morphological criteria and treated with Neomycin to select for cells reactivating the endogenous Sox2 gene. Undifferentiated miPSCs formed colonies very similar to murine embryonic stem cells (ESCs) ( Fig. 1a ), expressing the endogenous Sox2 gene ( Fig. 1b ). In vitro , the pluripotent state of miPSCs was validated by alkaline phosphatase (AP) activity ( Fig. 1c ) and by the expression of non-viral ESC marker genes such as Nanog , Oct4 , Sox2 , Klf4 , SSEA-1 ( Fig. 1d–f,j ). Moreover, upon embryoid bodies (EBs) formation, the presence of cells belonging to the three embryonic layers was confirmed by immunostaining for βIIITubulin (ectoderm), alpha smooth muscle actin (αSMA) (mesoderm) and forkhead box protein A2 (Foxa2) (endoderm) ( Fig. 1g–i ). In vivo , the generation of chimeric mice after blastocyst injection ( Fig. 1k ), and the formation of teratomas upon miPSCs transplantation into testes of SCID beige mice, provided further proof of the pluripotency of our miPSCs. Histological examination of tumours revealed the presence of tissues originating from the three germinal layers ( Fig. 1l–o ). 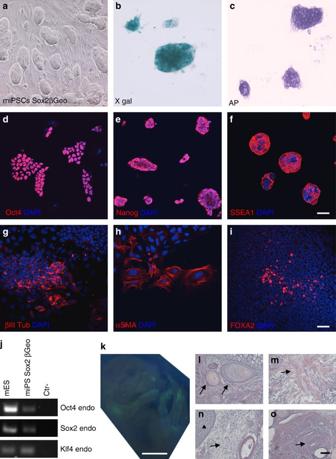Figure 1: Mouse induced pluripotent stem cells (miPSCs) generation and characterization. (a,b) miPSCs derived from the reprogramming of E14.5 C57Bl/6 Sox2βgeo/βgeoknock-in mouse embryo fibroblasts (miPSCs Sox2βgeo) (a) express a βgeo cassette under the control of Sox2 promoter that gives cell resistance to neomycin and the ability to be recognized by X-gal staining (b). (c–f) Immunochemistry for AP (c), Oct4 (d), Nanog (e) and SSEA-1 (f). Scale bar, 50 μm. (g–i) Immunostaining on differentiated miPSCs Sox2βgeo for βIIITubulin (ectoderm) (g), smooth muscle actin alpha (α-SMA; mesoderm) (h) and forkhead box protein A2 (FOXA2; endoderm) (i). Scale bar, 50 μm. (j) PCR analysis showing the activation of the endogenous pluripotency related genes:Oct4endo 224 bp;Sox2endo 297 bp; andKlf4endo 711 bp. (k) Blastocyst injection of GFP-positive miPSC Sox2βgeo generates chimeric mice. Scale bar, 5 mm. (l–o) Haematoxylin and Eosin staining on teratoma shows differentiated structures from all three germ layers. Immature epithelium (ectoderm) (l, arrows), muscle (mesoderm) (m, arrow), cartilage (mesoderm) (n, arrowhead), neural ectoderm (ectoderm) (n, arrow), glands (endoderm) (o, arrow).Scale bar, 1 mm. Figure 1: Mouse induced pluripotent stem cells (miPSCs) generation and characterization. ( a , b ) miPSCs derived from the reprogramming of E14.5 C57Bl/6 Sox2 βgeo/βgeo knock-in mouse embryo fibroblasts (miPSCs Sox2βgeo) ( a ) express a βgeo cassette under the control of Sox2 promoter that gives cell resistance to neomycin and the ability to be recognized by X-gal staining ( b ). ( c – f ) Immunochemistry for AP ( c ), Oct4 ( d ), Nanog ( e ) and SSEA-1 ( f ). Scale bar, 50 μm. ( g – i ) Immunostaining on differentiated miPSCs Sox2βgeo for βIIITubulin (ectoderm) ( g ), smooth muscle actin alpha (α-SMA; mesoderm) ( h ) and forkhead box protein A2 (FOXA2; endoderm) ( i ). Scale bar, 50 μm. ( j ) PCR analysis showing the activation of the endogenous pluripotency related genes: Oct4 endo 224 bp; Sox2 endo 297 bp; and Klf4 endo 711 bp. ( k ) Blastocyst injection of GFP-positive miPSC Sox2βgeo generates chimeric mice. Scale bar, 5 mm. ( l – o ) Haematoxylin and Eosin staining on teratoma shows differentiated structures from all three germ layers. Immature epithelium (ectoderm) ( l , arrows), muscle (mesoderm) ( m , arrow), cartilage (mesoderm) ( n , arrowhead), neural ectoderm (ectoderm) ( n , arrow), glands (endoderm) ( o , arrow).Scale bar, 1 mm. Full size image Generation of miPSC-NPCs from Sox2βGeo miPSCs A stable population of NPCs was derived from miPSCs Sox2βGeo ( Fig. 2 )—thereafter referred as miPSC-NPCs—as previously described [13] . Briefly, miPSCs Sox2βGeo, when plated in serum-free media, generated rosette-like structures, the hallmark of neuroepithelial differentiation. After 3–4 passages in neural precursors medium, cells were able to support neural progenitor proliferation, and additional split allowed us to purify an adherent homogeneous population of NPCs with a typical elongated bipolar morphology, end feet and oval nuclei ( Fig. 2a ). Cells were labelled in vitro using a third generation lentiviral vector encoding for GFP protein. More than 80% of the cells were labelled with this method ( Fig. 2b ). The neural stem cell identity of miPSC-NPCs was confirmed by the expression of the neural stem cell markers Nestin, Sox2, Olig2, Vimentin, BLBP, GLAST and Mash1 ( Fig. 2c–h ). Accordingly, miPSC-NPCs were able to self-renew over an extended period of time ( Fig. 2i ) and gave rise to neurons, astrocytes and oligodendrocytes when exposed to differentiating conditions ( Fig. 2j–l ) [14] , [15] , [16] . In conclusion, miPSC-NPCs met all the requirements of bona fide NPCs. 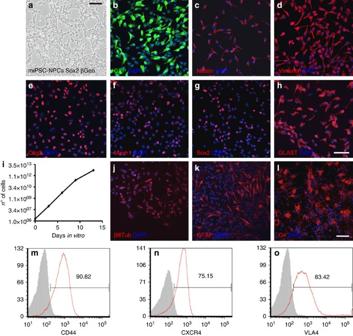Figure 2: Neural conversion of miPSC Sox2βgeo. (a) Bright field image of miPSC-NPCs obtained from miPSC Sox2βgeo. Scale bar, 50 μm. (b) GFP expression on miPSC-NPCs upon LV infection. Scale bar, 50 μm. (c–h) Immunostaining for Nestin (c), Vimentin (d), Olig2 (e), Mash1 (f), Sox2 (g) and GLAST (h). Scale bar, 50 μm. (i) Growth curve of miPSC-NPC. (j–l) Differentiation of miPSC-NPCs in three neural-derived cell populations, neurons (j), astrocytes (k) and oligodendrocytes (l). Scale bar, 50 μm. (m–o) Expression of the adhesion molecule CD44 (m), the chemokine receptor CXCR4 (n) and the integrin VLA-4 (o) onin vitrocultured miPSC-NPCs analysed by flow-activated cell sorting (FACS). Grey line represents the isotype control, whereas red line indicates the stained cells. Figure 2: Neural conversion of miPSC Sox2βgeo. ( a ) Bright field image of miPSC-NPCs obtained from miPSC Sox2βgeo. Scale bar, 50 μm. ( b ) GFP expression on miPSC-NPCs upon LV infection. Scale bar, 50 μm. ( c – h ) Immunostaining for Nestin ( c ), Vimentin ( d ), Olig2 ( e ), Mash1 ( f ), Sox2 ( g ) and GLAST ( h ). Scale bar, 50 μm. ( i ) Growth curve of miPSC-NPC. ( j – l ) Differentiation of miPSC-NPCs in three neural-derived cell populations, neurons ( j ), astrocytes ( k ) and oligodendrocytes ( l ). Scale bar, 50 μm. ( m – o ) Expression of the adhesion molecule CD44 ( m ), the chemokine receptor CXCR4 ( n ) and the integrin VLA-4 ( o ) on in vitro cultured miPSC-NPCs analysed by flow-activated cell sorting (FACS). Grey line represents the isotype control, whereas red line indicates the stained cells. Full size image miPSC-NPC treatment promotes functional recovery of EAE mice miPSC-NPCs were intrathecally transplanted into mice suffering from myelin oligodendrocyte glycoprotein (MOG) peptide 35–55-induced EAE at the peak of the disease (17.96±1.53 days post immunization (dpi)). Given the safety concerns related to the clinical translation of iPSC therapy [17] , we first analysed both CNS and peripheral organs from transplanted mice at 3 and 6 months after the cell injection and we did neither observe any toxicity nor tumour formation associated to miPSC-NPC treatment ( Supplementary Fig. S1 ). At 40 dpi, miPSC-NPC-treated EAE mice significantly ameliorated compared with sham- and MEF-treated mice ( Fig. 3a , Supplementary Fig. S2 ). Moreover, the inhibitory effect of miPSC-NPCs on EAE was specific and could not be obtained by other neural cells as there was no difference between astrocyte-transplanted and sham-treated groups in terms of clinical severity ( Supplementary Fig. S2 , Table 1 ). The therapeutic effect of miPSC-NPCs persisted up to the end of the follow-up: at 80 dpi, miPSC-NPC-treated mice reached an average EAE score of 1.0 (tail paralysis), while sham-treated mice reached an average score of 2.0 (hind limb paresis) ( Fig. 3a ). The clinical amelioration was paralleled by histopatological evidence of the reduction of demyelinated areas and axonal damage ( Fig. 3b–d ). Differentially expressed genes (DEG) analysis of the transcriptional profile associated with miPSC-NPC treatment of EAE mice found 428 differentially expressed probes (174 upregulated and 254 downregulated probes versus sham-treated group, Fig. 4a , right circle and Supplementary Data 1 ). Interestingly, among the 428 miPSC-NPC-related hits, 184 (~43%) appeared also among the EAE-related transcripts. Notably, out of 184 probes, 182 (50 upregulated and 132 downregulated) were expressed in miPSC-NPC spinal cord at levels similar to those measured in the spinal cord of naive animals (Venn diagram in Fig. 4a ). Accordingly, unsupervised hierarchical clustering based on the 184 common probes classified the miPSC-NPC group along with the naive group ( Fig. 4b ), providing the molecular evidence that the therapeutic effects exerted by transplanted miPSC-NPCs counterbalanced the EAE-associated transcriptional changes. 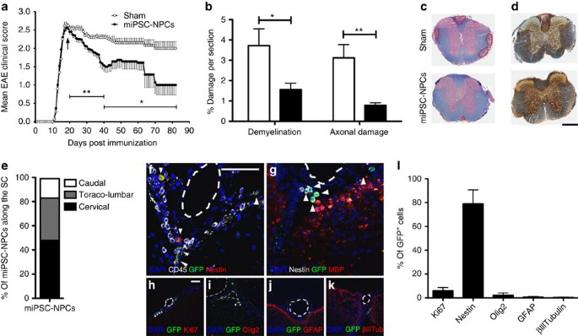Figure 3: Intrathecally transplanted miPSC-NPCs improve disease severity in EAE mice while remaining undifferentiated within perivascular spinal cord areas. (a) EAE clinical score of miPSC-NPC- (black dots) and sham-treated mice (white dots). Each point represents the mean disease score of at least 10 mice per group (±s.e.m.); two-way ANOVA; *P<0.05; **P<0.01. (b) Quantification of spinal cord demyelination and axonal damage at 80 dpi in miPSC-NPC- (black bars) versus sham-treated (white bars) EAE mice (N=6 per group). Data (mean values ±s.e.m.) represent the percentage of damage. Student’st-test; *P<0.05; **P<0.01. (c,d) Representative images of spinal cord sections stained with Luxol Fast Blue (c) and Bielschowsky (d). Red dotted lines represent areas of damage. Scale bar, 200 μm. (e) Quantitative analysis of the localization of miPSC-NPCs upon transplantation into EAE mice (N=3). (f–k) Immunostaining for CD45, MBP, Nestin, Ki67, Olig2, GFAP, βIII tubulin and GFP shows accumulation of transplanted cells (arrowheads) within perivascular spinal cord damaged areas. Dotted lines represent vessels. Nuclei are visualized with DAPI. Scale bars, 50 μm. (l) Percentage (±s.e.m.) of the miPSC-NPCs expressing the different neural differentiation markers upon transplantation into EAE mice; the majority of transplanted miPSC-NPCs remained undifferentiated. (N=3 mice per group). Figure 3: Intrathecally transplanted miPSC-NPCs improve disease severity in EAE mice while remaining undifferentiated within perivascular spinal cord areas. ( a ) EAE clinical score of miPSC-NPC- (black dots) and sham-treated mice (white dots). Each point represents the mean disease score of at least 10 mice per group (±s.e.m. ); two-way ANOVA; * P <0.05; ** P <0.01. ( b ) Quantification of spinal cord demyelination and axonal damage at 80 dpi in miPSC-NPC- (black bars) versus sham-treated (white bars) EAE mice ( N =6 per group). Data (mean values ±s.e.m.) represent the percentage of damage. Student’s t -test; * P <0.05; ** P <0.01. ( c , d ) Representative images of spinal cord sections stained with Luxol Fast Blue ( c ) and Bielschowsky ( d ). Red dotted lines represent areas of damage. Scale bar, 200 μm. ( e ) Quantitative analysis of the localization of miPSC-NPCs upon transplantation into EAE mice ( N =3). ( f – k ) Immunostaining for CD45, MBP, Nestin, Ki67, Olig2, GFAP, βIII tubulin and GFP shows accumulation of transplanted cells (arrowheads) within perivascular spinal cord damaged areas. Dotted lines represent vessels. Nuclei are visualized with DAPI. Scale bars, 50 μm. ( l ) Percentage (±s.e.m.) of the miPSC-NPCs expressing the different neural differentiation markers upon transplantation into EAE mice; the majority of transplanted miPSC-NPCs remained undifferentiated. ( N =3 mice per group). Full size image Table 1 Clinical characteristics of C57BL/6 EAE mice transplanted intrathecally with miPSC-NPCs, murine fibroblasts and murine astrocytes. 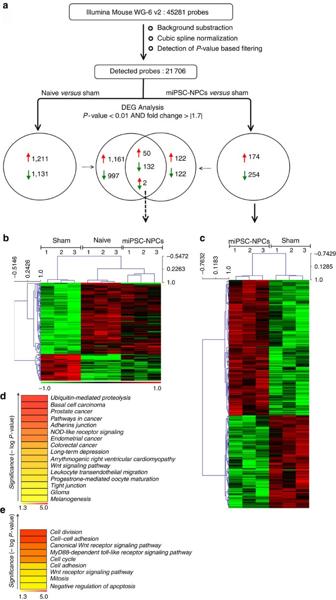Figure 4: Spinal cord transcriptomics in naive mice and miPSC-NPC- or sham-treated EAE mice. (a) Workflow of transcriptome analysis showing the differential expression between miPSC-NPC versus sham-treated EAE mice and naive mice versus sham-treated EAE mice. (b) Unsupervised hierarchical sample clustering based on 184 DEG common to the miPSC-NPC- versus sham-treated EAE mice and naive mice versus sham-treated EAE mice comparisons. (c) Unsupervised sample clustering based on 428 DEG between miPSC-NPC- and sham-treated EAE mice. (d) Significantly enriched KEGG pathways within the transcriptional profile from miPSC-NPC versus sham-treated EAE mice. (e) Significantly enriched biological processes in Gene Ontology. The colour gradient ranging from yellow to orange indicates the increasing statistical significance. Full size table Figure 4: Spinal cord transcriptomics in naive mice and miPSC-NPC- or sham-treated EAE mice. ( a ) Workflow of transcriptome analysis showing the differential expression between miPSC-NPC versus sham-treated EAE mice and naive mice versus sham-treated EAE mice. ( b ) Unsupervised hierarchical sample clustering based on 184 DEG common to the miPSC-NPC- versus sham-treated EAE mice and naive mice versus sham-treated EAE mice comparisons. ( c ) Unsupervised sample clustering based on 428 DEG between miPSC-NPC- and sham-treated EAE mice. ( d ) Significantly enriched KEGG pathways within the transcriptional profile from miPSC-NPC versus sham-treated EAE mice. ( e ) Significantly enriched biological processes in Gene Ontology. The colour gradient ranging from yellow to orange indicates the increasing statistical significance. Full size image miPSC-NPCs persist undifferentiated within perivascular infiltrates To further investigate the mechanism sustaining the neuroprotective effect of miPSC-NPC transplantation, we then analysed the tissue distribution of transplanted miPSC-NPCs in EAE mice. At 40 dpi, 1% of transplanted miPSC-NPCs localized within the entire neuraxis of EAE mice and distributed with a concentration gradient from the injection site to the caudal end of the CNS ( Fig. 3e ). Transplanted cells were found almost exclusively around subpial vessels where perivascular inflammatory infiltrates ( Fig. 3f ) and myelin damage were visible ( Fig. 3g ). The vast majority (79%) of transplanted cells maintained an undifferentiated phenotype (round morphology) and expressed nestin ( Fig. 3f,g,l ); only a small fraction displayed neuronal and glial differentiation markers—for example, Olig2 (2,2%), GFAP (0,6%), βIIITubulin (0,3%)—and the 6% of them proliferated ( Fig. 3h–l ). We attributed the miPSC-NPC pathotropism toward inflammatory lesions to the constitutive expression of chemotactic molecules such as CD44, VLA-4 and CXCR4 ( Fig. 2m–o ), as previously shown also for adult NPCs [6] , [7] , [18] , [19] , [20] . miPSC-NPCs restrain demyelination and promote remyelination Despite the lack of differentiation of transplanted cells into myelin-forming cells, the significant reduction of demyelination in the spinal cord of miPSC-NPC transplanted mice prompted us to further analyse the cellular characteristics of damaged areas. Within the demyelinating lesions of miPSC-NPC-treated EAE mice, we found an increased number of both proliferating Ki67 + /Olig2 + OPCs (0.69±0.19 versus 1.48±0.22 cells per field) ( Fig. 5a–c ) and mature CC1 + oligodendrocytes (4132±796.4 versus 2027±241.9 cells mm −2 ) ( Fig. 5d–f ). At the same time, we also found a reduction of apoptotic mature CC1 + /Caspase3 + oligodendrocytes ( Fig. 5g–i ) (9.17±3.08 versus 27.21±3.49% of cells). 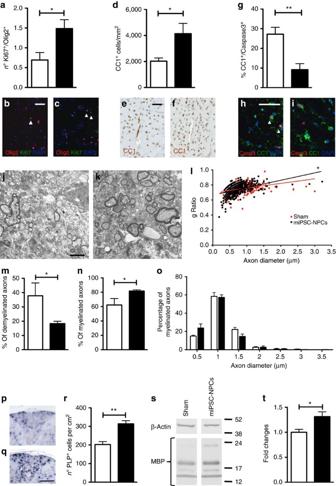Figure 5: miPSC-NPC transplantation restrains myelin damage and promote remyelination in EAE mice. (a–c) Quantification of Olig2+/Ki67+OPCs in the posterior column of the spinal cord from sham- (white bar) versus miPSC-NPC- (black bar) treated EAE mice (a) (N=6 mice per group). Representative images from sham- (b) versus miPSC-NPC- (c) treated EAE mice. (d–f) Quantification of the density of CC1+mature oligodendrocytes in the posterior columns of the spinal cord from sham- (white bar) versus miPSC-NPC- (black bar) treated EAE mice (d) (N=6 mice per group). Representative images from sham- (e) and miPSC-NPC-treated EAE mouse (f). (g–i) Quantification of the number of apoptotic CC1+mature oligodendrocytes in the spinal cord from sham- (white bar) versus miPSC-NPC (black bar) treated EAE mice (g) (N=6 mice per group). Representative images from sham- (h) and miPSC-NPC-treated EAE mouse (i). Scale bars, 50 μm. Arrowheads show double-positive cells. Data in panels (a,d,g) are expressed as mean (±s.e.m.). Student’st-test; *P<0.05; **P<0.01. (j,k) Electron micrographs representing a damaged spinal cord section from sham- (j) and miPSC-NPC (k) treated EAE mice. Scale bar, 2 μm. (l) Quantification of thegratios in miPSC-NPC (black) and sham- (red) treated EAE mice; data have been generated from more than 500-myelinated axons per group (N=3 mice per group) and show a significant increase of remyelinated fibres in miPSC-NSC-transplanted mice (Student’st-test;P=0.04). (m,n) Quantification of the percentage of demyelinated (m) and myelinated (n) axons in miPSC-NPC- (black) and sham- (white) treated EAE mice (N=3 mice per group). Data are expressed as mean (±s.e.m.). (o) Distribution of myelinated fibres in function of their diameter in miPSC-NPC (black bars) and sham- (white bars) treated EAE mice. (N=3 mice per group). Data are expressed as mean (±s.e.m.). (p–r) Representative images of DIG-basedin situhybridization for PLP-DM20 mRNA performed in spinal cord sections from sham- (p) versus miPSC-NPC-treated (q) EAE mice. Scale bar, 100 μm. (r) Quantification of the number of PLP-DM20+cells in the posterior column of the spinal cord from sham- (white bar) versus miPSC-NPC- (black bar) treated EAE mice (N=3 mice per group). Data are expressed as mean (±s.e.m.). (s,t) Western blot analysis for MBP in the spinal cord from sham- versus miPSC-NPC-treated EAE mice; blots are representative of three independent experiments (n). Quantification of the expression levels of MBP in the spinal cord from sham- (white bars) versus miPSC-NPC- (black bars) treated EAE mice (o). Data are expressed as mean (±s.e.m.).N= at least 3 mice per group. Student’st-test and Mann–Whitney test; *P<0.05; **P<0.005. Figure 5: miPSC-NPC transplantation restrains myelin damage and promote remyelination in EAE mice. ( a – c ) Quantification of Olig2 + /Ki67 + OPCs in the posterior column of the spinal cord from sham- (white bar) versus miPSC-NPC- (black bar) treated EAE mice ( a ) ( N =6 mice per group). Representative images from sham- ( b ) versus miPSC-NPC- ( c ) treated EAE mice. ( d – f ) Quantification of the density of CC1 + mature oligodendrocytes in the posterior columns of the spinal cord from sham- (white bar) versus miPSC-NPC- (black bar) treated EAE mice ( d ) ( N =6 mice per group). Representative images from sham- ( e ) and miPSC-NPC-treated EAE mouse ( f ). ( g – i ) Quantification of the number of apoptotic CC1 + mature oligodendrocytes in the spinal cord from sham- (white bar) versus miPSC-NPC (black bar) treated EAE mice ( g ) ( N =6 mice per group). Representative images from sham- ( h ) and miPSC-NPC-treated EAE mouse ( i ). Scale bars, 50 μm. Arrowheads show double-positive cells. Data in panels ( a , d , g ) are expressed as mean (±s.e.m.). Student’s t -test; * P <0.05; ** P <0.01. ( j , k ) Electron micrographs representing a damaged spinal cord section from sham- ( j ) and miPSC-NPC ( k ) treated EAE mice. Scale bar, 2 μm. ( l ) Quantification of the g ratios in miPSC-NPC (black) and sham- (red) treated EAE mice; data have been generated from more than 500-myelinated axons per group ( N =3 mice per group) and show a significant increase of remyelinated fibres in miPSC-NSC-transplanted mice (Student’s t -test; P =0.04). ( m , n ) Quantification of the percentage of demyelinated ( m ) and myelinated ( n ) axons in miPSC-NPC- (black) and sham- (white) treated EAE mice ( N =3 mice per group). Data are expressed as mean (±s.e.m.). ( o ) Distribution of myelinated fibres in function of their diameter in miPSC-NPC (black bars) and sham- (white bars) treated EAE mice. ( N =3 mice per group). Data are expressed as mean (±s.e.m.). ( p – r ) Representative images of DIG-based in situ hybridization for PLP-DM20 mRNA performed in spinal cord sections from sham- ( p ) versus miPSC-NPC-treated ( q ) EAE mice. Scale bar, 100 μm. ( r ) Quantification of the number of PLP-DM20 + cells in the posterior column of the spinal cord from sham- (white bar) versus miPSC-NPC- (black bar) treated EAE mice ( N =3 mice per group). Data are expressed as mean (±s.e.m.). ( s , t ) Western blot analysis for MBP in the spinal cord from sham- versus miPSC-NPC-treated EAE mice; blots are representative of three independent experiments ( n ). Quantification of the expression levels of MBP in the spinal cord from sham- (white bars) versus miPSC-NPC- (black bars) treated EAE mice ( o ). Data are expressed as mean (±s.e.m.). N = at least 3 mice per group. Student’s t -test and Mann–Whitney test; * P <0.05; ** P <0.005. Full size image Furthermore, ultrastructural analysis revealed a better preservation of myelin and axonal integrity ( Fig. 5j,k ) and a significant ( t- test P =0.04) increase of remyelinated axons in miPSC-NPC compared with sham-treated EAE mice ( Fig. 5l ). These latter results were paralleled by a significant decrease of demyelinated axons ( Fig. 5m ) and increase of myelinated axons ( Fig. 5n ) in miPSC-NPC compared with sham-treated EAE mice; a finding not depending from axon diameter ( Fig. 5o ). Finally, increased numbers of pro-myelinating PLP-DM20 + OPCs (313.7±16.79 versus 202.5±15.73 cells mm −2 ) ( Fig. 5p–r ) as well as increased levels of myelin basic protein (MBP) were found in the spinal cord tissue of miPSC-NPC versus sham-treated EAE mice ( Fig. 5s,t ); thus, further supporting an ongoing process of remyelination. Taken together, these results indicate that miPSC-NPC treatment preserves not only the viability but also the functionality of OPCs and mature oligodendrocytes, as these endogenous cells resulted capable of promoting remyelination and preservation of axonal integrity. Inflammation fosters miPSC-NPC-mediated OPC protection via LIF Given the propensity to maintain an undifferentiated phenotype upon in vivo transplantation, we postulated that miPSC-NPCs exerted the pro survival effect on OPCs and mature oligodendrocytes by releasing soluble trophic molecules [7] , [21] . Thus, we exposed in vitro OPCs to the medium obtained from miPSC-NPCs pre conditioned or not in vitro with TNFα and IFNγ ( Fig. 6a ); these latter two pro-inflammatory cytokines were used to mimic the inflamed tissue microenvironment in which transplanted miPSC-NPCs exerted their therapeutic functions as we previously showed [6] . After 5 days in culture, we found a significant increase of both OPCs and mature oligodendrocytes—as indicated by the increased number of O4 + cells (47.3±6.3% versus 26.9±4.09%), MBP + cells (17.1±1.2% versus 5.1±3.1%) and O4 + /Ki67 + cells (5.3±0.7% versus 0.3±0.2%)—in cultures treated with the TNFα/IFNγ pre conditioned medium compared to cultures treated with non-conditioned medium ( Supplementary Fig. S3a–e ). This finding suggested that miPSC-NPCs, upon inflammatory stimuli, secrete soluble factors with a trophic effect on both OPCs and mature oligodendrocytes. We next analysed which soluble molecule could be responsible for the trophic effect. Among several trophic factors tested, only the expression of LIF resulted markedly increased when miPSC-NPCs were challenged with TNFα/IFNγ ( Fig. 6b ). As a confirmation of LIF causative role, we found that anti-LIF antibody was able to inhibit OPC proliferation (of 5.3±0.7% versus 2.8±0.9% of O4 + /Ki67 + ) and differentiation into mature MBP + oligodendrocytes (17.1±1.2% versus 5.7±2.1%) as well as to reduce both OPCs and oligodendrocyte viability (47.3±6.2% versus 5.3±0.7% of O4 + cells) when added to the TNFα/IFNγ pre conditioned miPSC-NPC media ( Fig. 6c–h ). Moreover, the effect on OPCs and oligodendrocytes exerted by miPSC-NPC medium pre conditioned with TNFα/IFNγ was mimicked by rLIF ( Fig. 6c–i ). Together these data indicate that inflammation drives miPSC-NPCs to support OPC and oligodendrocyte survival and differentiation through the secretion of LIF. 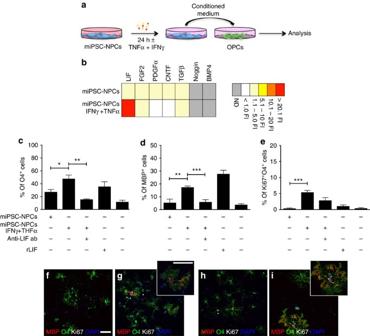Figure 6: LIF secreted by miPSC-NPCs conditioned with pro-inflammatory cytokines promotes OPC proliferation and differentiation. (a) Schematic representation of thein vitroexperimental design. (b) Semi-quantitative RT–PCR analysis of mRNA levels of pro-myelinating factor genes expressed by miPSC-NPCs pre conditioned or not with TNFα and IFNγ (ND=not detectable; FI=fold increase). (c–e) Quantification of the total number of O4+(c), MBP+(d) and O4+/Ki67+(e) cells per microscopic field. An anti-LIF neutralizing antibody (anti-LIF ab) and the recombinant LIF (rLIF) have been added to OPC cultures when indicated. Data represent the mean (± s.e.m.) of three independent experiments compared with non-treated culture. Student’st-test; *P<0.05; **P<0.01; ***P<0.001; NS, not significant. (f–i) Representative images of OPCs cultured in non-conditioned medium (f), conditioned medium (g), conditioned medium with anti-LIF ab (h) and medium with rLIF (i). Triple staining for MBP (red), O4 (green) and Ki67 (white, arrowheads). Nuclei are counterstained with DAPI (Blue). Scale bars, 50 μm. Figure 6: LIF secreted by miPSC-NPCs conditioned with pro-inflammatory cytokines promotes OPC proliferation and differentiation. ( a ) Schematic representation of the in vitro experimental design. ( b ) Semi-quantitative RT–PCR analysis of mRNA levels of pro-myelinating factor genes expressed by miPSC-NPCs pre conditioned or not with TNFα and IFNγ (ND=not detectable; FI=fold increase). ( c – e ) Quantification of the total number of O4 + ( c ), MBP + ( d ) and O4 + /Ki67 + ( e ) cells per microscopic field. An anti-LIF neutralizing antibody (anti-LIF ab) and the recombinant LIF (rLIF) have been added to OPC cultures when indicated. Data represent the mean (± s.e.m.) of three independent experiments compared with non-treated culture. Student’s t -test; * P <0.05; ** P <0.01; *** P <0.001; NS, not significant. ( f – i ) Representative images of OPCs cultured in non-conditioned medium ( f ), conditioned medium ( g ), conditioned medium with anti-LIF ab ( h ) and medium with rLIF ( i ). Triple staining for MBP (red), O4 (green) and Ki67 (white, arrowheads). Nuclei are counterstained with DAPI (Blue). Scale bars, 50 μm. Full size image LIF exerts a trophic effect on endogenous oligodendrocytes We next investigated whether LIF was also responsible of the in vivo effect observed upon miPSC-NPC transplantation in EAE mice. We first showed that transplanted miPSC-NPCs located within perivascular inflammatory infiltrates—and therefore sensing the inflammatory environment—produce LIF; a finding confirmed at both protein and mRNA levels via immunofluorescence and in situ hybridization ( Fig. 7a,b ). Then, we observed an increased level of the phosphorylated form of the signal transducer and activator of transcription-3 (pSTAT3), a well-known downstream LIF pathway signalling molecule [22] , in the spinal cord of miPSC-NPC- compared with sham-treated EAE mice ( Fig. 7c,d ) and an increased number of CC1 + oligodendrocytes expressing pSTAT3 ( Fig. 7e,f ). Finally, miPSC-NPC transplanted EAE mice treated with a continuous intrathecal infusion of the neutralizing anti-LIF antibody showed a significantly more severe EAE (mean score post-treatment 3.2±0.3 versus 2.2±0.2) ( Fig. 7g ). Interestingly, although the number of inflammatory infiltrates at 30 dpi was superimposable among groups ( Fig. 7h ), a significant increase in the percentage of demyelinated areas (1.9±0.2% versus 1.15±0.1%) ( Fig. 7i ), in the number of apoptotic mature CC1 + /Caspase3 + oligodendrocytes (11.29±5.49% versus 32.58±0.48%) ( Fig. 7j ) as well as a reduction of mature CC1 + oligodendrocytes (1,086±248.0 versus 4,398±1,860 cells mm −2 ) ( Fig. 7k ) was found in EAE mice treated with iPSC-NPCs plus anti-LIF ab versus mice treated with miPSC-NPCs alone. Collectively, these results indicate an activation of the LIF pathway in vivo upon miPSC-NPC transplantation, and confirm that LIF is necessary for the clinical amelioration and myelin preservation induced by miPSC-NPC transplantation. 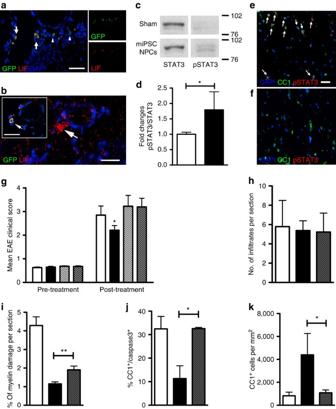Figure 7: LIF secreted by transplanted miPSC-NPCs promotesin vivoa trophic effect on endogenous oligodendrocytes. (a) Representative immunostaining for LIF and GFP of perivascular inflammatory areas of the spinal cord from miPSC-NPC-treated EAE mice. Nuclei are counterstained with DAPI. Scale bar, 50 μm. (b) Representative images of radioactive-basedin situhybridization for LIF mRNA; LIF+cell are located near perivascular inflammatory areas (arrows). In the inset, co-localization of LIF mRNA expressing and LIF-producing cells is shown in adjacent tissue sections. Scale bars, 50 μm. (c) Representative immunoblot quantifying pSTAT3 and STAT3 in the spinal cord from sham- versus- miPSC-NPC-treated EAE mice. (d) Ratio between immunoblot intensity of tyrosine-phosphorylated STAT3 (pSTAT3) versus STAT3 in miPSC-NPC- (black bars) versus sham-treated EAE mice (white bars) (N=3 mice per group). Data are expressed as mean (±s.e.m.). Student’st-test; *P< 0,05. (e,f) Immunostaining for pSTAT3 and CC1 in miPSC-NPC (e) versus sham-treated (f) EAE mice (scale bar, 50 μm). (g) EAE score (mean±s.e.m.) before and after the treatment with sham (white bars), miPSC-NPCs (black bars), sham plus anti-LIF ab (light grey bars) and miPSC-NPCs plus anti-LIF ab (dark grey bars). One-way ANOVA (N=5 per group), *P<0.05. (h,i) Quantification of the number of inflammatory infiltrates (h) and percentage of myelin damage (i) in the spinal cord of EAE mice 10 days after sham (white bars), miPSC-NPCs (black bars) or miPSC-NPCs plus anti-LIF ab (dark grey bars) treatments (N=3 mice per group). Data are expressed as mean (±s.e.m.). Student’st-test; **P<0.005. (j,k) Quantification of the density of CC1+mature oligodendrocytes (j) and of the number of apoptotic CC1+/Caspase3+mature oligodendrocytes (k) in the posterior columns of the spinal cord of EAE mice 10 days after sham (white bar), miPSC-NPC- (black bar) or miPSC-NPCs plus anti-LIF ab (dark grey bars) treatments (N=3 mice per group). Data are expressed as mean (±s.e.m.). Student’st-test; *P<0.05. Figure 7: LIF secreted by transplanted miPSC-NPCs promotes in vivo a trophic effect on endogenous oligodendrocytes. ( a ) Representative immunostaining for LIF and GFP of perivascular inflammatory areas of the spinal cord from miPSC-NPC-treated EAE mice. Nuclei are counterstained with DAPI. Scale bar, 50 μm. ( b ) Representative images of radioactive-based in situ hybridization for LIF mRNA; LIF + cell are located near perivascular inflammatory areas (arrows). In the inset, co-localization of LIF mRNA expressing and LIF-producing cells is shown in adjacent tissue sections. Scale bars, 50 μm. ( c ) Representative immunoblot quantifying pSTAT3 and STAT3 in the spinal cord from sham- versus- miPSC-NPC-treated EAE mice. ( d ) Ratio between immunoblot intensity of tyrosine-phosphorylated STAT3 (pSTAT3) versus STAT3 in miPSC-NPC- (black bars) versus sham-treated EAE mice (white bars) ( N =3 mice per group). Data are expressed as mean (±s.e.m.). Student’s t -test; * P < 0,05. ( e , f ) Immunostaining for pSTAT3 and CC1 in miPSC-NPC ( e ) versus sham-treated ( f ) EAE mice (scale bar, 50 μm). ( g ) EAE score (mean±s.e.m.) before and after the treatment with sham (white bars), miPSC-NPCs (black bars), sham plus anti-LIF ab (light grey bars) and miPSC-NPCs plus anti-LIF ab (dark grey bars). One-way ANOVA ( N =5 per group), * P <0.05. ( h , i ) Quantification of the number of inflammatory infiltrates ( h ) and percentage of myelin damage ( i ) in the spinal cord of EAE mice 10 days after sham (white bars), miPSC-NPCs (black bars) or miPSC-NPCs plus anti-LIF ab (dark grey bars) treatments ( N =3 mice per group). Data are expressed as mean (±s.e.m.). Student’s t -test; ** P <0.005. ( j , k ) Quantification of the density of CC1 + mature oligodendrocytes ( j ) and of the number of apoptotic CC1 + /Caspase3 + mature oligodendrocytes ( k ) in the posterior columns of the spinal cord of EAE mice 10 days after sham (white bar), miPSC-NPC- (black bar) or miPSC-NPCs plus anti-LIF ab (dark grey bars) treatments ( N =3 mice per group). Data are expressed as mean (±s.e.m.). Student’s t -test; * P <0.05. Full size image miPSC-NPC trophic effect limits CNS-confined inflammation Oligodendrocyte death occurring as a consequence of EAE results in the generation of partially disrupted myelin debris that act as endogenous inflammatory stimuli capable of exacerbating the CNS-confined inflammatory process [23] . As a direct consequence of this phenomenon axonal regeneration and remyelination are inhibited [24] and BBB permeability altered [25] . Transcriptomics and functional annotation data—indicating that transcripts involved in cell survival/death processes were differentially regulated in miPSC-NPC transplanted EAE mice at 40 dpi ( Fig. 4d,e and Supplementary Data 1 )—and the observed reduction of apoptotic mature oligodendrocytes in transplanted mice ( Fig. 5g–i ) prompted us to evaluate whether or not the neuroprotective effect exerted by miPSC-NPCs might have also indirectly affected the overall neuroinflammatory reaction. We first analysed the inflammatory burden in miPSC-NPC and sham-treated mice at different time points after EAE onset. At 30 dpi, we found that the number and the composition of the CNS inflammatory infiltrates—including enchephalitogenic Th1 and Th17 cells—were similar between the two groups ( Figs 8a–o and 9a,c–e ). Moreover, real-time PCR analysing the expression of molecules usually associated with blood derived beneficial (M2) monocytes/macrophages [26] , [27] —that is, Arginase1, CD206, YM-1, IL4Rα and TGFβ—were similarly expressed in the whole-spinal cord of sham- versus miPSC-NPC-treated EAE mice ( Fig. 8p–t ). 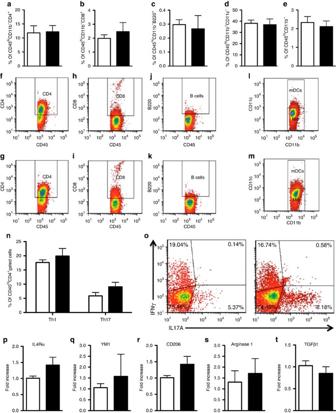Figure 8: Inflammatory CNS-infiltrate cellular characteristics in EAE mice transplanted with miPSC-NPCs. (a–e) Flow cytometry of CNS-infiltrating blood-borne inflammatory cells in sham versus miPSC-NPC-treated EAE mice at 30 dpi (N=4 mice per group). CNS-infiltrating leukocytes are gated as CD45hiCD11b−cells, T-cell subpopulations as CD4+(a) and CD8+(b), B cells as CD45hiCD11b−B220+(c), macrophages (MΦ) as CD45hiCD11b+CD11c−(d), and dendritic cells (mDC) as CD45hiCD11b+CD11c+(e). Percentages have been calculated on the total CD45-gated cells (± s.d.). (f–m) Representative plots of all CNS-infiltrating inflammatory cells. Sham-treated EAE mice are represented in the upper panels (f,h,j,l), whereas miSPC-NPC-treated EAE mice in the lower panels (g,i,k,m). (n) Quantification of encephalitogenic Th1 and Th17 cells derived from sham versus miPSC-NPC-treated EAE mice at 30 dpi. Percentages have been calculated on the total CD45hiCD4+gated cells (±s.d.). (o) Representative plots of CNS-infiltrating Th1 and Th17 cells population, identified based on their production of IFNγ and IL-17A, respectively, on sham-treated (left) and miPSC-NPC (right)-treated EAE mice. (p–t) Real-time PCR-based expression analysis of M2-type monocytes/macrophages-related genes in the spinal cord tissue from miPSC-NPC- (black bars) and sham-treated (white bars) EAE mice (N=5 mice per group). Results are expressed as fold increase over basal expression level in sham-treated mice (mean±s.e.m.). Figure 8: Inflammatory CNS-infiltrate cellular characteristics in EAE mice transplanted with miPSC-NPCs. ( a – e ) Flow cytometry of CNS-infiltrating blood-borne inflammatory cells in sham versus miPSC-NPC-treated EAE mice at 30 dpi ( N =4 mice per group). CNS-infiltrating leukocytes are gated as CD45 hi CD11b − cells, T-cell subpopulations as CD4 + ( a ) and CD8 + ( b ), B cells as CD45 hi CD11b − B220 + ( c ), macrophages (MΦ) as CD45 hi CD11b + CD11c − ( d ), and dendritic cells (mDC) as CD45 hi CD11b + CD11c + ( e ). Percentages have been calculated on the total CD45-gated cells (± s.d.). ( f – m ) Representative plots of all CNS-infiltrating inflammatory cells. Sham-treated EAE mice are represented in the upper panels ( f , h , j , l ), whereas miSPC-NPC-treated EAE mice in the lower panels ( g , i , k , m ). ( n ) Quantification of encephalitogenic Th1 and Th17 cells derived from sham versus miPSC-NPC-treated EAE mice at 30 dpi. Percentages have been calculated on the total CD45 hi CD4 + gated cells (±s.d.). ( o ) Representative plots of CNS-infiltrating Th1 and Th17 cells population, identified based on their production of IFNγ and IL-17A, respectively, on sham-treated (left) and miPSC-NPC (right)-treated EAE mice. ( p – t ) Real-time PCR-based expression analysis of M2-type monocytes/macrophages-related genes in the spinal cord tissue from miPSC-NPC- (black bars) and sham-treated (white bars) EAE mice ( N =5 mice per group). Results are expressed as fold increase over basal expression level in sham-treated mice (mean±s.e.m.). 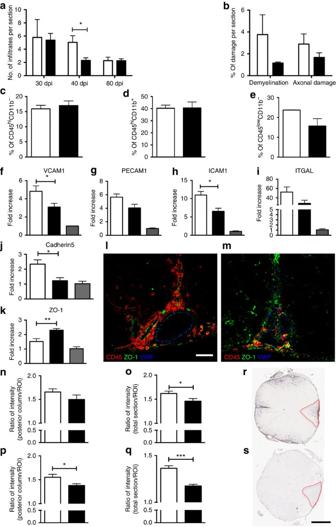Figure 9: miPSC-NPC transplantation limits the CNS entry of blood-borne inflammatory cells by preserving BBB integrity and permeability. (a) Quantification of the number of inflammatory infiltrates in the spinal cord tissue from miPSC-NPC (black bars) and sham-treated (white bars) EAE mice at 30, 40 and 80 dpi. Analyses are performed on hematoxylin and eosin staining. Data are expressed as mean (±s.e.m.). Student’st-test; *P<0.05. (b) At 30 dpi, quantification of Luxol fast blue (demyelination) and Bielschowsky (axonal damage) staining in the spinal cord tissue from miPSC-NPC- (black bars) versus sham-treated (white bars) EAE mice. Data are expressed as mean (±s.e.m.). Student’st-test (N=3 mice per group); *P<0.05. (c–e) FACS analysis of CNS-infiltrating subpopulations of inflammatory mononuclear cells at 30 dpi in the spinal cord tissue from miPSC-NPC (black bars) and sham-treated (white bars) EAE mice. CNS-invading populations are identified on the basis of the level of the expression of CD45 and CD11b and numbers of CNS-invading lymphocytes (CD45hiCD11b−) (c), myeloid cells (CD45hiCD11b+) (d) and microglia (CD45lowCD11b+) (e) were quantified. The percentage of each CNS-infiltrating cell subpopulation is calculated on the total CD45-gated cells (mean±s.e.m.). (f–k) Real-time PCR-based expression analysis in the spinal cord tissue from miPSC-NPC- (black bars) and sham-treated (white bars) EAE mice; naive untreated mice are also represented (grey bars). Results are expressed as fold increase over basal expression level in naive mice (mean±s.e.m.); Student’st-test (N=3 mice per group); *P<0,05, **P<0.005. (l,m) Immunostaining for ZO-1, CD45 and von Willebrand Factor (vWF) in sham- (l) and miPSC-NPC- (m) treated EAE mice. Scale bar,50 μm. (n–q) Quantification of IgG extravasation in the spinal cord of miPSC-NPC (black bars) or sham (white bars)-treated EAE mice at 30 dpi (n,o) and at 40 dpi (p,q) (mean ±s.e.m.). Bars inn,prepresent the ratio of IgG signal intensity measured in the spinal cord posterior columns versus an arbitrary region used as normalizer (that is, ROI) at 30 dpi (n) and 40 dpi (m). Bars ino,qrepresent the ratio between the the entire spinal cord area versus ROI at 30 dpi (o) and 40 dpi (q). Student’st-test (N=3 mice per group); *P<0,05, ***P<0,001. (r,s) Immunohistochemistry for IgG extravasation in sham- (r) versus miPSC-NPC-treated (s) EAE mice. Broken red lines indicate the posterior columns. Scale bar, 200 μm. Full size image Figure 9: miPSC-NPC transplantation limits the CNS entry of blood-borne inflammatory cells by preserving BBB integrity and permeability. ( a ) Quantification of the number of inflammatory infiltrates in the spinal cord tissue from miPSC-NPC (black bars) and sham-treated (white bars) EAE mice at 30, 40 and 80 dpi. Analyses are performed on hematoxylin and eosin staining. Data are expressed as mean (±s.e.m.). Student’s t -test; * P <0.05. ( b ) At 30 dpi, quantification of Luxol fast blue (demyelination) and Bielschowsky (axonal damage) staining in the spinal cord tissue from miPSC-NPC- (black bars) versus sham-treated (white bars) EAE mice. Data are expressed as mean (±s.e.m.). Student’s t -test ( N =3 mice per group); * P <0.05. ( c – e ) FACS analysis of CNS-infiltrating subpopulations of inflammatory mononuclear cells at 30 dpi in the spinal cord tissue from miPSC-NPC (black bars) and sham-treated (white bars) EAE mice. CNS-invading populations are identified on the basis of the level of the expression of CD45 and CD11b and numbers of CNS-invading lymphocytes (CD45 hi CD11b − ) ( c ), myeloid cells (CD45 hi CD11b + ) ( d ) and microglia (CD45 low CD11b + ) ( e ) were quantified. The percentage of each CNS-infiltrating cell subpopulation is calculated on the total CD45-gated cells (mean±s.e.m.). ( f – k ) Real-time PCR-based expression analysis in the spinal cord tissue from miPSC-NPC- (black bars) and sham-treated (white bars) EAE mice; naive untreated mice are also represented (grey bars). Results are expressed as fold increase over basal expression level in naive mice (mean±s.e.m. ); Student’s t -test ( N =3 mice per group); * P <0,05, ** P <0.005. ( l , m ) Immunostaining for ZO-1, CD45 and von Willebrand Factor (vWF) in sham- ( l ) and miPSC-NPC- ( m ) treated EAE mice. Scale bar,50 μm. ( n – q ) Quantification of IgG extravasation in the spinal cord of miPSC-NPC (black bars) or sham (white bars)-treated EAE mice at 30 dpi ( n , o ) and at 40 dpi ( p , q ) (mean ±s.e.m.). Bars in n , p represent the ratio of IgG signal intensity measured in the spinal cord posterior columns versus an arbitrary region used as normalizer (that is, ROI) at 30 dpi ( n ) and 40 dpi ( m ). Bars in o , q represent the ratio between the the entire spinal cord area versus ROI at 30 dpi ( o ) and 40 dpi ( q ). Student’s t -test ( N =3 mice per group); * P <0,05, *** P <0,001. ( r , s ) Immunohistochemistry for IgG extravasation in sham- ( r ) versus miPSC-NPC-treated ( s ) EAE mice. Broken red lines indicate the posterior columns. Scale bar, 200 μm. Full size image At the same time point, demyelination and axonal loss were significantly reduced in miPSC-NPC-treated EAE mice ( Fig. 9b ). Contrariwise, at 40 dpi, inflammation was significantly less pronounced in miPSC-NPC versus sham-treated EAE mice ( Fig. 9a ). At 80 dpi, inflammation subsided in both groups of EAE mice ( Fig. 9a ). As the kinetic of the inflammatory burden in transplanted EAE mice was compatible with the working hypothesis, we further assessed which of the inflammatory components was involved in this process. We focused on BBB not only because an increase of BBB permeability is a key event leading to CNS infiltration of blood-borne inflammatory cells [28] but also because pathway analysis revealed an enrichment in sham-treated versus transplanted EAE mice of transcripts belonging to two BBB-related pathways, that is, tight-junctions and adherent-junctions, and one pathway related to CNS migration of inflammatory blood-borne mononuclear cells, that is, leukocyte transendothelial migration ( Fig. 4d ). Quantitative RT–PCR analysis confirmed a return to baseline values of mRNA levels of vascular cell adhesion protein 1 (VCAM1), platelet/endothelial cell adhesion molecule 1 (PECAM1), intercellular adhesion molecule 1 (ICAM1) and integrin (alpha L) lymphocyte function-associated antigen 1 (ITGAL1), Chaderin-5 upon miPSC-NPC transplantation in EAE mice ( Fig. 9f–j ). On the other hand, expression level of ZO-1—a molecule necessary to seal the BBB and reduce permeability and cellular extravasation [29] —was increased upon miPSC-NPC treatment compared with the baseline level ( Fig. 9k–m ). As all these findings indicated that miPSC-NPC transplantation might have preserved BBB integrity, we next assessed BBB permeability. A significant reduction of IgG extravasation was observed in miPSC-NPC versus sham-treated EAE mice as early as 30 dpi ( Fig. 9n,o ); a reduction which was further increased at 40 dpi ( Fig. 9p–s ). All together these results suggest that the miPSC-NPC-mediated trophic effect on the viability of endogenous CNS-resident myelin-forming cells, preserves BBB permeability and integrity and limits the continuous CNS recruitment of encephalitogenic blood-borne inflammatory cells. Here we show that transplantation of miPSC-NPCs represents a therapeutically efficacious strategy in inflammatory demyelinating disorders. The therapeutic effect was not due to a cell replacement mechanism [30] , [31] , [32] , but to the in situ release of neuroprotective molecules by transplanted cells. We found that neuroinflammation occurring in EAE mice was capable to attract miPSC-NPCs to the site of myelin damage and to instruct such cells to secrete LIF that, in turn, promoted endogenous myelin-forming cell survival and functionality. This mechanism, alternative to cell replacement, renders miPSC-NPCs a suitable candidate for cell therapy in multifocal inflammatory demyelinating disease, such as MS. Indeed, although it was shown that myelin-forming cells could be generated from iPSCs [3] or directly reprogrammed from somatic cells [33] , [34] , it was not known the therapeutic potential of these cells when transplanted into a myelin hostile inflammatory environment, such as that characterizing MS. Given that myelin damage is often accompanied by reactive inflammation or it is caused, as in our experimental setting, by primary inflammation, it is mandatory to find a population of stem/progenitor cells that is able to exert its neuroprotective effect within an inflammatory environment. Although the pro survival function of LIF is not surprising as there are several in vitro but also in vivo data suggesting that such factor promotes OPC and mature oligodendrocyte survival via a STAT3-mediated intracellular signalling pathway [35] , [36] , [37] , it is surprising that the miPSC-NPC-mediated therapeutic effect was very rapid and efficient. Our results suggest that this finding can be attributed to a primary neuroprotective effect of miPSC-NPC secreted LIF leading to a secondary anti-inflammatory effect. As a matter of fact, the neurprotective effect of LIF, induced a less pronounced damage of myelin-forming cells and this was sufficient to reduce the overall inflammatory burden, which has been variably shown to be dependent on the amount of tissue destruction [38] . The restraint of the inflammatory process, in turn, provoked a reduction of the BBB leakage that eventually inhibited CNS extravasation of encephalitogenic blood-borne inflammatory mononuclear cells [39] , [40] . Whether or not iPSC-NPC transplantation might favour—directly or indirectly—CNS infiltration of blood derived (alternatively activated) beneficial M2 monocytes/macrophages can be only envisaged at this stage; interestingly, we observed a slight increased expression of genes related to the M2 lineage in the spinal cord of miPSC-NPC compared with sham-treated EAE mice. Finally, we cannot exclude that the neuroprotective effect exerted by miPSC-NPCs could be amplified by other cell types known to secrete LIF (that is, astrocytes). Moreover, other factors may have influenced the LIF-mediated effect on oligodendrocytes, as a similar effect was recently observed for mesenchimal stem cell transplantation via hepatocyte growth factor secretion [41] . In conclusion, although proposing a novel mechanism of action our results further expand the therapeutic potential of iPSC-derived NPCs and suggest that preservation of myelin-forming cells integrity might represent a valid anti-inflammatory strategy to promote tissue repair in immune-mediated demyelinating disorders. Lentiviral Vector (LV) production A LV expressing the Oct4 , Sox2 and Klf4 genes from a single cistron (named reprogramming LV—rep.LV) and a LV expressing ubiquitously eGFP (named LV.eGFP) were used in this study. LVs were prepared as previously described [42] . Briefly, 293T cells were co-transfected by calcium phosphate precipitation with the following four plasmids: the transfer vector plasmid (32 μg), being either the transfer vector containing the expression cassette for the reprogramming genes or the transfer vector expressing eGFP; the pMD.Lg/pRRE packaging plasmid (12.5 μg); the pMD2.VSV-G envelope-encoding plasmid (9 μg); (iv) pCMV-Rev (6.25 μg). Viral vectors were concentrated by ultra-centrifugation and transduced cells were analysed by FACS (FACSCalibur, Becton Dickinson Immunocytometry Systems). Fibroblast culture and miPSC generation MEFs were isolated from E14.5 C57BL/6 Sox2 βgeo/βgeo knock-in mice embryos [12] . These mice contain a βgeo cassette that encodes for β-galactosidase activity (lacZ) as well as G418 resistance. Fibroblasts were cultured in Dulbecco’s modified Eagle’s medium (DMEM) high glucose (Euroclone), 15% fetal bovine serum (FBS; Euroclone), 2 mM L -glutamine (Euroclone), and 1% penicillin/streptomycin (Invitrogen). For iPSC generation, 10 5 fibroblasts were infected with the rep.LV in DMEM 10% FBS and 4 μg ml −1 of polybrene. After 1 week, the transduced fibroblasts were plated on a feeder layer of Mitomycin C (Sigma-Aldrich) treated MEFs (1.2 × 10 6 cells per 10 cm dish) in DMEM supplemented with 15% FBS, 2 mM L -glutamine, 0.1 mM nonessential amino acids, 1 mM sodium pyruvate, 0.1 mM β-mercaptoethanol, 5 mg ml −1 penicillin, 100 mg ml −1 streptomycin and 10 3 U ml −1 LIF (Chemicon International). Medium was changed every day and colonies started to appear 20 days later. At around day 40, colonies were transferred to a new feeder layer Neomicin resistant and pluripotent colonies were selected thanks to their resistance to G418 treatment (Neomicin analogue). Subsequently, miPSCs clones were split by Trypsin treatment every 2 days at a 1 to 6 dilution. Pluripotency of miPSCs have been assessed by RT–PCR using a set of primers previously described [13] : Oct4 endo TCTTTCCACCAGGCCCCCGGCTC TGCGGGCGGACATGGGGAGATCC (224 bp); Sox2 endo TAGAGCTAGACTCCGGGCGATGA TTGCCTTAAACAAGACCACGAAA (297 bp); Klf4 endo GCGAACTCACACAGGCGAGAAACC TCGCTTCCTCTTCCTCCGACACA (711 bp). AP staining Direct AP activity was analysed using the NBT/BCIP (AP) blue substrate (Roche), according to the manufacturer’s guidelines. LacZ staining was performed on cultured cells after fixation for 3 min at 4 °C with 4% paraformaldehyde (PFA) and then incubated for 12 h at 37 °C in X-Gal reaction buffer (PBS, 35 mM potassium ferrocyanide, 35 mM potassium ferricyanide, 2 mM MgCl2, 0.02% nonidet P-40 (NP-40), 0.01% Na deoxycholate) containing 1 mg ml −1 5-bromo-4-chloro-3-indolyl-β- D -galactopyranoside (X-Gal; Sigma-Aldrich). Embryoid body differentiation miPSCs were dissociated by Trypsin (Invitrogen) incubation for 20 min at 37 °C; EBs were generated by culturing the cells in suspension on bacterial dish (Sterlin) at 10 5 cells ml −1 in mES medium without LIF. After 3 days, EBs were plated on 0.1% gelatin (Sigma-Aldrich) coated tissue culture dishes and cells were analysed 4 days after. Chimera generation After injection of 8–10 Sox2βGeo miPSCs in each E3.5 blastocyst isolated from C57Bl/6 mice, blastocysts were transferred into E2.5 pseudo-pregnant CD1 females, and chimeras were analysed at embryonic day 13–14 by GFP fluorescence. Teratoma formation SCID beige mice were anaesthetized with 140 ml of anaesthetic solution containing 12.5% ketamine and 6.25% xylazine in 0.9% saline solution before starting surgery. Testes were exposed and 1 × 10 6 miPSCs resuspended in 10 ml of PBS were injected within the right testis. The successful rate of teratoma generation was of 100% and after 6 weeks mice were killed. Tumours were removed and processed for light microscopy. Paraffin-embedded tissue sections were stained for hematoxylin and eosin. Derivation and culture of miPSC-NPCs miPSC-NPCs were obtained from Sox2βgeo miPSCs following the published protocol [13] . miPSC-NPCs were cultured in adhesion in NPC proliferation medium: Euromed-N medium (Euroclone), N 2 supplement (Invitrogen), 20 ng ml −1 EGF (Peprotech Inc.) and 20 ng ml −1 FGF-2 (Peprotech Inc.). For routine passaging, miPSC-NPCs were dissociated to single-cell suspension with Acutase (Sigma) and split 1:4 or 1:5 every 2–3 days. Differentiation of miPSC-NPCs miPSC-NPCs were differentiated into astrocytes, neurons and oligodendrocytes as previously described [13] , [15] , [16] . Briefly, astrocytes were obtained by adding 5% of FBS to the medium culture. For neural differentiation, miPSC-NPCs were exposed to B27, then plated on laminin-coated glass coverslips in the presence of decreasing concentrations of FGF-2 while gradually adding brain-derived neurotrophic factor up to 30 ng ml −1 in 10–15 days. To obtain oligodendrocytes, miPSC-NPCs were plated on glass coverslips pre-treated with polyornithine and laminin. Oligodendrocyte differentiation required an intermediate glial precursor stage, supported by the platelet-derived growth factor (PDGF)α and the mitogen forskolin, followed by growth factor withdrawal and addition of triiodothyronine (T3) and ascorbic acid (AA) for 1 week to promote terminal differentiation into the oligodendrocyte lineage. EAE induction Chronic-relapsing EAE was induced in 6–8 weeks C57Bl/6 female mice (Charls River) by subcutaneous immunization with MOG 35–55 peptide (200 μg per mouse) in incomplete Freund’s adjuvant containing 8 mg ml −1 Mycobacterium tuberculosis (strain H37Ra; Difco). Mice were i.v. injected with 500 ng of pertussis toxin (Sigma) the day of the immunization and 2 days later. Body weight and clinical score (0=healthy; 1=limp tail; 2=ataxia and/or paresis of hindlimbs; 3=paralysis of hindlimbs and/or paresis of forelimbs; 4=tetraparalysis; 5=death) was recorded daily [6] . All procedures involving animals were performed according to the guidelines of the Animal Ethical Committee of our Institute (IACUC). miPSC-NPC transplantation Six to eight weeks C57Bl/6 female mice (Charls River) were anaesthetized with 12.5% ketamine and 6.25% xylazine in 0.9% saline solution. miPSC-NPCs, murine fibroblasts and murine astrocytes (1 × 10 6 cells per mouse diluted in 10 μl) were transplanted by stereotaxic injection into cisterna magna of EAE mice at the peak of the disease (4 days after disease onset). Age- and sex-matched sham (PBS)-treated EAE mice were sued as controls. MEFs were obtained by C57Bl/6 mouse pups as described above, while mouse primary astrocytes were prepared from newborn mice following published procedures [43] . Briefly, forebrains were collected from newborn C57Bl/6 mouse pups and carefully freed of meninges, chopped into 0.25-mm sections and dissociated by a mild trypsinization procedure and gentle mechanical disruption with a Pasteur pipette. The cells were seeded into poly- L -lysine (10 μg ml −1 )-coated 175-cm 2 flasks at the density of 4 × 10 4 cells cm −2 and grown at 37 °C in a 92% air–8% CO 2 humidified atmosphere in DMEM (Invitrogen) containing 0.45-μm filtered, 10% FBS (Invitrogen), 2 mM glutamine (BioWhittaker, Verviers, Belgium), penicillin (100 U ml −1 ) and streptomycin (100 μg ml −1 ). The medium was replaced after 24 h and then every 3 days. After about 10 days in vitro , primary cultures were vigorously shaken to detach microglia and oligodendrocytes growing on top of the astrocytic layer. The remaining adherent cells were detached with trypsin (0.25%)/EDTA, resuspended in fresh medium and reseeded on poly- L -lysine-coated plastic surfaces. Purity of mouse astrocyte cultures was checked by GFAP staining and was >95%. At the time of killing—which occurred at different time points after immunization (30, 40 and 80 dpi)—at least 10 mice per group were anaesthetized and transcardially perfused with saline solution followed by 4% PFA. Brains, spinal cords and peripheral organs (heart, lungs, liver, spleen, gut and kidney) were removed and processed for light and electron microscopy. LIF neutralization in EAE mice Subcutaneous osmotic minipumps (ALZET, model 1007) were implanted in EAE mice after sham or miPSC-NPC treatment. Two microgram per day of LIF neutralizing antibody (R&D) were dissolved in PBS and administered for 7 days intracerebroventricularly to EAE mice using a brain catheter (Brain Infusion Kit 3, ALZET) connected to the subcutaneously implanted osmotic minipump. Stereotaxic apparatus was used to determine the exact location of the brain catheter inside the lateral ventricle (from bregma, 0.3 mm anterior, 0.8 lateral). Neuropathological analysis Paraffin-embedded tissue sections were stained for hematoxylin and eosin, Luxol fast blue and Bielshowsky silver impregnation to detect inflammatory infiltrates, demyelination and axonal loss, respectively. The number of perivascular inflammatory infiltrates was calculated as the mean number of inflammatory infiltrates per spinal cord section. Six animals per group were analysed. For analysis of demyelination and axonal damage, paraffin-embedded, adjacent serial transverse spinal cord sections (5 μm) were stained with Luxol fast blue/periodic-acid Schiff staining and Bielschowsky silver impregnation. Tissue damage was marked with ImageJ and expressed as the percentage of damage area on the entire spinal cord section. At least 5 animals per group (miPSC-NPCs and Sham) were analysed and 12 to 20 different rostro-caudal sections were marked per animal. Statistical significance was assessed by unpaired Student’s t -test. Immunofluorescence and immunohistochemistry Cells in culture and tissues (20 μm) were fixed with 4% PFA in phosphate buffer solution (PBS) pH 7.2 and tissues were cryoprotected for at least 24 h in 30% Sucrose (Sigma) in PBS at +4 °C. Coronal brain and spinal cord sections (20 μm) and fixed cells were incubated with blocking solution (PBS 1x, FBS 10%, BSA 1 mg ml −1 and Triton 0.1%) for 1 h and then primary antibodies were applied in the same solution over night at +4 °C. The following primary antibodies were used: mouse α-OCT4 (1:50, Santa Cruz Biotechnology); rabbit α-Nanog (1:200, Millipore); mouse α-SSEA3 (1:150, Millipore); Foxa2; αSMA; mouse α-Vimentin (1:200, Abcam); rabbit α-Mash1 (1:200, Chemicon); GLAST; rabbit α-Sox2 (1:100, Millipore); α-Ki67 (1:1,000, Novocastra); rabbit α-TuJ1 (1:1,000, Covance); rabbit α-Olig2 (1:200, Chemicon); mouse α-Olig2 (1:300, Chemicon); mouse α-GFAP (1:1,000, Chemicon); rabbit α-GFAP (1:1,500, Dako); mouse α-O4 (1:100, Millipore); rabbit α-NG2 (1:200, Santa Cruz); mouse α-Nestin (1:100, BD Pharmagen); chicken α-GFP (1:300, Abcam); rabbit α-pSTAT3 (1:200, Cell Signalling); rabbit α-STAT3 (1:200, Cell Signalling); rat α-MBP (1:200, Chemicon); goat α-LIF (1:50, R&D); mouse α-APC (1:100, Calbiochem); mouse α-ZO-1 (1:150, ); rabbit α-von Willebrand Factor (1:1000, Abcam); rat α-CD45 (1:100, BD Pharmagen); rabbit α-caspase3 clived (1:200, Cell Signalling). Appropriate fluorophore-conjugated secondary antibodies (Alexa Fluor 488, 546, 405 and 633, Molecular Probes) or alternatively the chromogen DAB (Vector Laboratories) were used for detection accordingly manufacturer’s instructions. Omission of the primary antibodies showed no specific staining. Nuclei were stained with 4′,6-diamidino-2-phenylindole (DAPI, Roche). Immunopositive cells within lesions were counted once the extent of the demyelination had been established with Luxol fast blue staining on adjacent sections. Microscopy was performed using Light (Olympus, BX51 equipped with × 4 and × 20 objectives) and confocal (Leica, SP5 equipped with × 20 and × 40 objectives) and images were analysed by using Leica LCS lite and Adobe Photoshop CS software (Adobe Systems Incorporated, CA 95110, USA). in situ hybridization Radioactive and DIG in situ hybridization were performed as follows [44] . Briefly, radioactive in situ hybridization was performed on 20 μm-thick spinal cord sections post-fixed 15 min in 4% PFA, washed three times in PBS and incubated in 0.5 mg ml −1 of Proteinase K (Roche) in 100 mM Tris-HCl (pH 8), 50 mM EDTA for 10 min at 30 °C. After a second 15 min fixation was done in 4% PFA, slices were then washed three times in PBS, once in H 2 O and then incubated in triethanolamine (Merk) 0.1 M (pH 8) for 5 min. Four hundred microlitre of acetic anhydride (Sigma) was added twice for 5 min. Finally, sections were rinsed in H2O for 2 min and air-dried. Hybridization was performed overnight at 60 °C with α-UTP-P33 (GE) LIF riboprobe at a concentration ranging from 10 6 to 10 7 counts per minute (c.p.m.). The day after, sections were rinsed in SSC 5X for 5 min then washed in formamide 50% (Sigma)-SSC 2X for 30 min at 60 °C. Slides were then incubated in ribonuclease-A (Roche) 20 mg ml −1 in 0.5 M NaCl, 10 mM Tris-HCl (pH 8), 5 mM EDTA 30 min at 37 °C, then washed in formamide 50% SSC 2X for 30 min at 60 °C and rinsed two times in SSC 2X. Finally, slides were dried using ethanol series. Lm1 (GE Healthcare Life Sciences, Milan, Italy) emulsion was applied in dark room, according manufacturer’s instructions. After 1 week, sections were developed in dark room, counterstained with DAPI and mounted with DPX (BDH) mounting solution. DIG in situ hybridization was performed as described for radioactive one. In details, PLP-DM20 riboprobe was synthesized using DIG RNA Labeling Mix (Roche). Hybridization was performed overnight at 60 °C with Digriboprobes. After last SSC 2X wash, slices were incubated in Tris-HCl 2 M, NaCl 5 M for 1 h at room temperature. Primary antibody α-Dig-POD (α-Dig conjugated with horse-radish peroxidase; 1:2,000, Roche) was added and incubated overnight at 4 °C. Sections were then washed with 0.1 M Tris-HCl pH=9.5, 0, 1 M NaCl, 50 mM MgCl 2 and subjected to BCIP (5-bromo-4-chloro-3-indolyl-phosphate)/NBT (nitro blue tetrazolium) for the colorimetric detection. PLP-DM20 riboprobe was kindly provided by Robin Franklin (Cambridge, UK) and LIF riboprobe was PCR generated based on NCBI Reference Sequence NM_001039537. Microphotographs of sections were digitalized in dark field light microscopy (Olympus BX51, and × 4 objective) by using a CCD camera (Leica). Images were analysed by using Adobe Photoshop CS. To confirm the specificity of the different RNA probes, sense strand RNA probes (showing no signal) were used as negative controls. Electron microscopy Mice were perfused as described above. Spinal cord tissue was removed and fixed with 2% (vol/vol) glutaraldehyde in 0.12 M phosphate buffer, post-fixed with 1% (wt/vol) osmium tetroxide and embedded in Epon (Fluka). Semithin (1 μm thick) and ultrathin (70–80 nm thick) sections were cut from the spinal cord. Semithin sections were stained with toluidine blue. For electron microscopy, ultrathin sections were stained with uranyl acetate and lead citrate and examined by electron microscopy (Leo 912 Omega) using a × 100 objective [45] . The percentage and the number of myelinated/demyelinated axons and G ratio measurements were performed on digitized non overlapping electron micrographs images. G ratios were determined by dividing the mean diameter of an axon without myelin by the mean diameter of the same axon with myelin. To determine the size distribution of myelinated fibres in the spinal cord, diameters of all fibres in at least 10 randomly chosen representative images were measured and binned based on their width. The number of myelinated and nonmyelinated axons were counted in at least ten randomly chosen representative images. All measurements were acquired on × 100 semithin section images. Immunoblotting Spinal cord tissue was collected from at least three saline perfused EAE mice per group and homogenized in a lysis buffer containing 2% SDS, 95 mM NaCl, 10 mM EDTA, 1 mM PMSF, 10 μg ml −1 aprotinin, 20 μM leupeptin, 1 mM orthovanadate and 2.5 mM sodium pyrophosphate in 25 mM Tris buffer (pH 7.4). Protein concentrations were determined by the BCA method (Pierce) [46] . Ten to 20 μg of protein for samples were fractionated by SDS–PAGE and blotted onto nitrocellulose (Protran Biosciences). After blocking in 4% milk in TBST (0.1% Triton X-100 in TBS), appropriate regions were incubated with specific primary antibody prepared in 5% BSA, 0.05% sodium azide in TBST and secondary antibodies and developed with the ECL western blotting Detection Reagent (GE Healthcare). Semi-quantitative western blot analysis was performed using ImageJ software. Raw data are shown in Supplementary Fig. S4 . Antibodies: mouse monoclonal α-MBP (SMI-94, SMI-99); rabbit α-phospho-STAT3 (1:200, Cell Signalling); rabbit α-STAT3 (1:200, Cell Signalling). OPC culture In our in vitro studies we used rat oligodendrocyte precursors following the myelinating oligodendrocyte coculture system developed by Chan et al . [47] This is a well established and used system that allows the preparation of a significant amount of pure OPCs. We purposely used rat oligodendrocytes in order to obtain enough pure cells for performing all the in vitro experiments. Thus, to avoid possible effects due to species’ differences, we have tested the effects of LIF and conditioned media also on rat OPCs prepared by differential immunopanning. Primary OPCs from P1 Sprague–Dawley rat cortices were grown over an astrocyte monolayer in DMEM, 10% FBS (Invitrogen). After 10 days, OPCs were separated by orbital shaking and immunopanned using anti Ran-2 and A2B5 (refs 47 , 48 ). Fifty thousand A2B5 + OPCs were plated on poly-lysin coated glass coverslips and kept in DMEM containing 10% FBS. The following day, medium was changed to SATO medium supplemented with proliferating (10 ng ml −1 FGF and 10 ng ml −1 PDGFα) or differentiating (30 ng ml −1 T3) growth factors or to conditioned SATO medium. Conditioned medium was obtained by the culture of 1 × 10 6 miPSC-NPCs in 5 ml of SATO for 24 h with or without inflammatory cytokines (10 ng ml −1 IFNγ and 15 ng ml −1 TNFα). For LIF neutralization, supernatant of miPSC-NPCs cultured with or without inflammatory cytokines was harvested at 24 h from miPSC-NPC cultures and supplemented with LIF neutralizing antibody (R&D) (0.5 μg ml −1 ). Recombinant LIF (rLIF) (1 ng ml −1 ) was added to SATO medium as positive control. At least four coverslips were subjected to each culture condition and three biological replicate were performed. In this culturing condition, differentiation of OPCs was quantified by counting the number of MBP + (that is, mature oligodendrocytes), O4 + (that is, OPCs and oligodendrocytes), and O4 + /Ki67 + (that is, OPCs) cells in at least 10 fields per the coverslip. RNA extraction and RT–PCR Total RNA was extracted from the spinal cord of minimum five mice per group and from cells using Trizol reagent (Invitrogen) and residual DNA was removed by treatment with 1 U DNase per 1 mg RNA (RQ1 RNase-free DNase, Promega) at 37 °C for 30 min according to manufacturer’s procedures. cDNA synthesis was performed by using ThermoScriptTM RT–PCR System (Invitrogen) and Random Hexamer (Invitrogen). mRNA levels were measured by real-time RT–PCR (Applied Biosystem, Invitrogen). The 2− ΔΔCT method was used to calculate relative changes in gene expression [49] . The following Applied Biosystem (Invitrogen) probes were used: LIF (Mm00434761_m1), FGF-2 (Mm00433287_m1), PDGF (Mm00833533_m1), CNTF (Mm00446373_m1), TGFβ (Mm03024053_m1), Noggin (Mm00476456_s1), BMP4 (Mm00432087_m1), Chaderin-5 (Cdh5) (Mm00486938_m1), ICAM (Mm00476227_m1), VCAM1 (Mm00449197_m1), PECAM1 (Mm01242584_m1), ITGAL (Mm00801807_m1), ZO-1 (Mm01320637_m1), Pten (Mm1212532_m1), IL4ra (Mm01275139_m1), YM-1 (Mm00657889_m1), CD206 (Mm00485148_m1), and Arg1 (Mm00475988_m1). Isolation of CNS-infiltrating mononuclear cells Ten days after the treatment, EAE mice were intracardially perfused with cold HBSS and spinal cords and hindbrains were collected. Tissues were homogenized with neural tissue dissociation kit according to the manufacturer’s procedures (Miltenyi Biotech). CNS-infiltrating mononuclear cells were isolated from discontinuous 30%:70% Percoll gradient [50] . Briefly, the homogenate was resuspended in 30% Percoll (Pharmacia, Piscataway, NJ), and underlaid with 70% Percoll. The gradients were centrifuged at 2,400 g at 24 °C for 20 min. CNS mononuclear cells were collected from the Percoll interface, washed and resuspended in FACS buffer (phenol red negative Hank’s BSS with 10% FBS) for further analysis. Flow-activated cytometric analysis For surface staining, CNS-infiltrating cells isolated form EAE mice or miPSC-NPCs were incubated with 5% fetal calf serum, 2% rat serum and 2.5 μg ml −1 rat anti-mouse Fc III/II receptor (CD16/CD32) blocking antibodies (BD Pharmingen) for 10 min at 4 °C and then stained for 30 min at 4 °C with the following directly conjugated monoclonal primary antibodies specific for mouse antigens: CD4 (RM4-5), CD11b (M1/70), CD11c (N418), CD45.2 (104), CD8 (Ly-2), CD45R/B220 (RA3-6B2), CD44 (IM/7) (BD Pharmingen), VLA-4 (PS/2; Abcam), CXCR4 (2B11; eBioscience). As negative control, we used florescence mix minus one colour for multiple staining and the corresponding isotype control for single staining. For intracellular cytokine staining, cells were stimulated for 6 h with phorbol 12-myristate 13-acetate (50 ng ml −1 ) and ionomycin (500 ng ml −1 ) in the presence of GolgiPlug (BD Pharmingen). Then, cells were stained for surface molecules, fixed and made permeable with a Cytofix/Cytoperm Plus kit (BD Bioscience) and stained with the following antibodies: IL-17A (TC11-18H10) and IFN-γ (XMG1.2) (all from BD Pharmingen). The cells were washed and analysed. Data were acquired with a Canto II flow cytometer (Becton Dickinson) and analyses were performed with DIVA or FCS Express V3 software. Microarray analysis Three mice per group (naive, miPSC-NPC-treated or sham-treated), at 40 dpi, were anaesthetized and transcardially perfused with RNase-free 0.9% saline containing 10 U ml −1 of heparin at 40 dpi. CNS was collected, and brain and spinal cord of each animal were separately homogenized in 1 ml of QIAzol Lysis Reagent (Qiagen, Valencia, CA, USA, #79306) using a rotor-stator homogenizer. RNA was extracted according to manufacturer instructions and their concentration was determined spectrophotometrically by A260 (Nanodrop-ND 1000, Nanodrop, Wilmington, DE, USA). cRNA amplification was performed using the Illumina TotalPrep RNA Amplification Kit (Ambion) and 1.5 μg of biotin-labelled cRNA of each sample was hybridized on Illumina MouseWG-6 v2 expression bead chip (Illumina). The array contained 45281 probes representing transcripts contained in the NCBI-Refseq, Riken, and Meebo databases. The raw data were background subtracted and cubic spine normalized using Illumina GenomeStudio software. Detection P -values reported by the GenomeStudio were used to estimate the amount of detected probes [51] , and a threshold of detection P -value<0.05 was applied for filtering. No outlier samples were found in principal component analysis and hierarchical sample clustering. Differential gene expression analysis were performed in the R-bioconductor platform and the empirical Bayes test was used as implemented in the LIMMA package [52] . DEG passed P -value<0.01 and ±1.7 fold change thresholds and were used for bioinformatical functional annotation. Pathway and Gene Onotology enrichment analyses were performed using the Genecodis tool [53] , with the enrichment criteria of at least three genes in one category and P -value<0.05, computed from χ 2 -test followed by Benjamini–Hochberg’s correction. Statistical analysis Statistical evaluations of RT–PCR data, immunoblot data, FACS data, EAE score and immunohistochemical analyses results were expressed as mean±s.e.m. Results were analysed using the unpaired Student’s t -test and two-way ANOVA for clinical score analysis. Mann–Whitney test was used when non parametric data have been compared and analysed. Analyses were performed using the Prism V5.0a software (Graph-Pad, San Diego, CA, USA). Statistical significance was accepted when * P <0.05, ** P <0.01, *** P <0.001. Accession codes: The MIAME-compliant microarray data have been deposited in the EBI ArrayExpress database under accession number E- MTAB-1546 . How to cite this article: Laterza, C. et al . iPSC-derived neural precursors exert a neuroprotective role in immune-mediated demyelination via the secretion of LIF. Nat. Commun. 4:2597 doi: 10.1038/ncomms3597 (2013).